The complete sequence of the smallest known nuclear genome from the microsporidianEncephalitozoon intestinalis The genome of the microsporidia Encephalitozoon cuniculi is widely recognized as a model for extreme reduction and compaction. At only 2.9 Mbp, the genome encodes approximately 2,000 densely packed genes and little else. However, the nuclear genome of its sister, Encephalitozoon intestinalis , is even more reduced; at 2.3 Mbp, it represents a 20% reduction from an already severely compacted genome, raising the question, what else can be lost? In this paper, we describe the complete sequence of the E. intestinalis genome and its comparison with that of E. cuniculi . The two species share a conserved gene content, order and density over most of their genomes. The exceptions are the subtelomeric regions, where E. intestinalis chromosomes are missing large gene blocks of sequence found in E. cuniculi . In the remaining gene-dense chromosome 'cores', the diminutive intergenic sequences and introns are actually more highly conserved than the genes themselves, suggesting that they have reached the limits of reduction for a fully functional genome. Microsporidia are a group of obligate intracellular parasites of agricultural and medical importance that are widely recognized as highly adapted fungi [1] , [2] , [3] , [4] , [5] , [6] . Their obligate intracellular lifestyle is characterized by a high degree of host dependence [7] , leading to, among other things, an extraordinary reduction in the number of genes encoded in their genomes. In addition to losing many genes, however, several microsporidian genomes have also evolved a very high gene density, partly by the shortening of the genes themselves, but more substantially by reducing their intergenic regions. In the most extreme cases, genes are tightly packed with intergenic spaces averaging just over 100 bp, and several protein-coding sequences physically overlap with their neighbours. The miniaturization of these genomes has affected not just form but also function, in particular leading to frequent overlaps between the mRNA transcripts of adjacent genes in many species [8] , [9] , [10] , [11] . Genome compaction has also seemingly affected the rate at which microsporidian parasites shuffle their genomes; hence, the order of genes is conserved, even between species separated by very large genetic distances [12] , [13] , despite the fact that the genes themselves are known to be evolving very rapidly at the sequence level. Overall, microsporidian nuclear genomes are the most reduced and compacted of any eukaryotic cell, including picoplankton and other obligately intracellular parasites such as Plasmodium , the agent of malaria. The model organism for these highly compacted genomes is the human parasite Encephalitozoon cuniculi , the completely sequenced genome of which is only 2.9 Mbp [3] . With approximately 2,000 genes, this genome is indeed strikingly reduced; however, this is not the smallest known microsporidian genome. The genome of the closely related species, E. intestinalis , has been estimated by pulsed field gel electrophoresis to be only 2.3 Mbp [14] , which corresponds to 600 kbp or 20% smaller than E. cuniculi . Given the already reduced nature of E. cuniculi , one wonders what else can be lost. At the extremes, either hundreds of genes were lost or the entire genome was even more radically compacted. Unfortunately, currently, no data exist on the nature of this smallest known nuclear genome to reveal what evolutionary forces might operate at the far end of the spectrum of genome reduction. In this study, we describe the complete genome sequence of E. intestinalis (ATCC 50506). A comparison between this genome and that of its sibling species, E. cuniculi , reveals that virtually all of the difference in genome size can be attributed to large subtelomeric regions that are present in E. cuniculi but absent from E. intestinalis . The remainder of the genome is relatively conserved in content, order and density, and indeed we find that the intergenic regions and the introns are remarkably well conserved at the sequence level, altogether suggesting that these chromosome 'cores' have reached a certain limit of reduction and additional substantial changes to them are likely to be difficult. General features of the E. intestinalis genome A total of 200 ng of E. intestinalis DNA was isolated from purified spores and used for Solexa sequencing, from which the entire genome was assembled de novo , resulting in an assembly of 137 scaffolds with an average coverage of 40×. PCR and Sanger sequencing were used to link the preliminary scaffolds and polish internal breaks, resulting in 11 large contigs homologous to the 11 chromosomes of E. cuniculi , with a total sequence of 2,191,783 Mbp, or >95% of the estimated 2.3 Mbp ( Fig. 1 ). 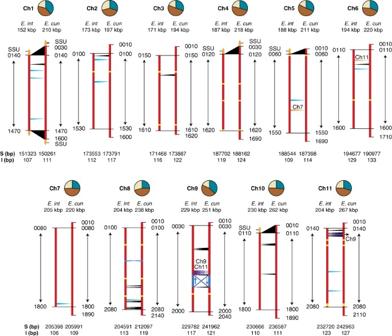Figure 1: Comparison between the chromosomes ofE. intestinalisandE. cuniculi. Comparison of the 11 chromosomes ofE. intestinalis(left side) andE. cuniculi(right side), with the total assembled size for each indicated below the name. Difference in the relative length of orthologous protein-coding genes is summarized in a pie chart above each chromosome. Blue, brown and beige colours represent the portion of proteins that are, respectively, shorter, identical or longer inE. intestinaliscompared withE. cuniculiorthologues. Chromosome 'cores' are shown in red and the size (S) and average intergenic regions (I) of each core are indicated under it. Gene rearrangements, inversions and events of gene losses and gains between species are shown as coloured triangles. Black triangles represent the location of genes absent fromE. intestinalis. Light blue rectangles represent the location of genes absent fromE. cuniculi. Yellow rectangles represent genes that were previously unannotated inE. cuniculithat have been identified by comparisons withE. intestinalis. In addition, it was evident for many other genes that the previous annotation used the wrong ATG codon. The newly annotated version of theE. cuniculigenome is available asSupplementary Data 1. Dark orange triangles represent genes duplicated and rearranged between chromosomes ofE. intestinalis(chromosome number shown above the rectangle). Dark violet arrows represent genes transposed from another chromosome (original chromosome number shown above the rectangle). Chromosomal inversions are shown in dark blue. SSU, small subunit ribosomal RNA gene. The E. intestinalis genome harbours the same complement of transfer RNAs and ribosomal RNAs as E. cuniculi and both genomes have a similar GC content ( Table 1 ). The subtelomeric regions of microsporidian chromosomes typically consist of a mixture of unique genes and repeated gene families, ending with a copy of the ribosomal RNA operon [3] , [15] . We found a 22-fold excess of ribosomal RNA operon in our assembly, suggesting that it is also located in the subtelomeric regions of all 11 chromosomes in E. intestinalis . In five cases, we linked the ribosomal RNA operon to the end of a chromosome assembly by PCR, representing all three subtelomeric regions known in E. cuniculi , plus two additional ones ( Fig. 1 ). Figure 1: Comparison between the chromosomes of E. intestinalis and E. cuniculi . Comparison of the 11 chromosomes of E. intestinalis (left side) and E. cuniculi (right side), with the total assembled size for each indicated below the name. Difference in the relative length of orthologous protein-coding genes is summarized in a pie chart above each chromosome. Blue, brown and beige colours represent the portion of proteins that are, respectively, shorter, identical or longer in E. intestinalis compared with E. cuniculi orthologues. Chromosome 'cores' are shown in red and the size (S) and average intergenic regions (I) of each core are indicated under it. Gene rearrangements, inversions and events of gene losses and gains between species are shown as coloured triangles. Black triangles represent the location of genes absent from E. intestinalis . Light blue rectangles represent the location of genes absent from E. cuniculi . Yellow rectangles represent genes that were previously unannotated in E. cuniculi that have been identified by comparisons with E. intestinalis . In addition, it was evident for many other genes that the previous annotation used the wrong ATG codon. The newly annotated version of the E. cuniculi genome is available as Supplementary Data 1 . Dark orange triangles represent genes duplicated and rearranged between chromosomes of E. intestinalis (chromosome number shown above the rectangle). Dark violet arrows represent genes transposed from another chromosome (original chromosome number shown above the rectangle). Chromosomal inversions are shown in dark blue. SSU, small subunit ribosomal RNA gene. Full size image Table 1 General characteristics of the genomes of E. intestinalis and other microsporidia. Full size table Coding capacity of the smallest nuclear genome The coding capacity and structure of the E. intestinalis genome were identified using manual annotation and compared against our own manually annotated version of the E. cuniculi genome (available as Supplementary Data 1 ) and the genomes of other microsporidian relatives [3] , [13] , [16] , [17] , [18] , [19] . Altogether, 1,833 protein-coding genes were identified in the assembly. If complete, this would result in a coding capacity that is almost 10% smaller than that of E. cuniculi , and the smallest identified in a eukaryote. The complexity of its proteome is, however, predicted to be very similar to that of other microsporidia ( Table 1 , Supplementary Table S1 ) because the majority of those genes found to be absent from E. intestinalis are hypothetical proteins or duplicates of genes that are present. Only 15 protein-coding genes with known function in E. cuniculi were found to be absent in E. intestinalis , whereas only four such genes were found in E. intestinalis but not in E. cuniculi . These did not correspond to whole pathways, but were instead a scattered representation of various functions ( Supplementary Data 2 ). Interestingly, 10 other hypothetical genes with no known function were also found in E. intestinalis but have no recognizable orthologue in E. cuniculi ; three of these are known from other microsporidia, whereas seven are exclusive to E. intestinalis ( Supplementary Data 2 ). Finally, 16 genes that were previously unannotated in E. cuniculi were identified on the basis of homology to E. intestinalis ( Supplementary Data 2 ), bringing the total number of protein-coding genes in E. cuniculi to 1,999 ( Table 1 ). This number, which is based on a direct comparison with that of E. intestinalis , is lower than previous estimates, even though several new genes were identified because a number of previously annotated open reading frames (ORFs) now seem to be spurious (see our own annotation of the E. cuniculi genome, available as Supplementary Data 1 ). Genome evolution along the chromosomes of E. intestinalis A comparison between E. intestinalis and E. cuniculi genomes revealed that their chromosome 'cores' are, with a few exceptions, completely colinear, despite significant divergence in sequence ( Fig. 1 ; see 'Methods' section for our definition of the chromosome 'cores'). Only two chromosomal inversions and two transpositions between chromosomes 9 and 11 were found, and two E. cuniculi genes were found to be duplicated and rearranged in E. intestinalis (an ABC transporter and a ubiquitin hydrolase). The average gene density of E. intestinalis (0.86 genes/kbp) was only fractionally higher than that of E. cuniculi (0.84 genes/kbp) and the two genomes share the same reduced complement of introns. The E. intestinalis genes and introns were themselves reduced in size only slightly more than those of E. cuniculi (on an average, proteins are 0.06% shorter in E. intestinalis , Table 1 ), whereas the intergenic regions are reduced by 3.6% ( Figs 1 and 2 and Table 1 ). Together with the slight reduction in the number of genes encoded within the chromosome 'cores' (1,819 of E. intestinalis as opposed to 1,830 in E. cuniculi when putative pseudogenes are not counted; Supplementary Data 2 ), reduction in the 'core' accounts for only about 34 kbp of the overall difference between the genome assemblies of E. intestinalis (95% assembled) and E. cuniculi (85% assembled), most of which is due to gene loss ( Fig. 2 ). 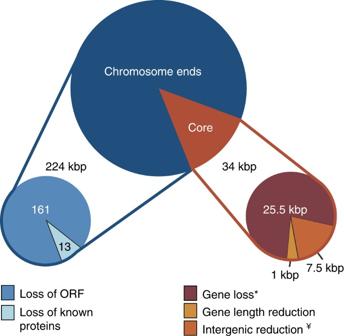Figure 2: Genome reduction inE. intestinalis. A comparison between the genome assembly ofE. intestinalis(>95% assembled) with the available assembly ofE. cuniculi(85% assembled) shows that the vast majority of genes that are absent inE. intestinalisare located at the chromosome ends inE. cuniculi(left,n=174, 161 ORFs and 13 genes of identified function,Supplementary Data 2). At the chromosome cores, gene losses and shortening of intergenic regions account for most of the reduction in size ofE. intestinalis, whereas reduction in gene length is negligible.*Includes their surrounding intergenic spaces.¥Calculations are based on orthologous intergenic regions only. Figure 2: Genome reduction in E. intestinalis . A comparison between the genome assembly of E. intestinalis (>95% assembled) with the available assembly of E. cuniculi (85% assembled) shows that the vast majority of genes that are absent in E. intestinalis are located at the chromosome ends in E. cuniculi (left, n =174, 161 ORFs and 13 genes of identified function, Supplementary Data 2 ). At the chromosome cores, gene losses and shortening of intergenic regions account for most of the reduction in size of E. intestinalis , whereas reduction in gene length is negligible. * Includes their surrounding intergenic spaces. ¥ Calculations are based on orthologous intergenic regions only. Full size image In contrast to the cores, the E. intestinalis subtelomeres that we identified in this study are substantially reduced compared with those of E. cuniculi . Only three such regions have been completely characterized in E. cuniculi (two on chromosome 1, one on chromosome 4). We characterized all three corresponding regions in E. intestinalis , as well as two additional examples on chromosomes 5 and 10 ( Fig. 3 ). These regions harbour a mixture of unique genes of known function in other organisms, hypothetical ORFs, and several members of a highly divergent Encephalitozoon -specific gene family (for example, DUF1609, DUF2463 or DUF1686) that seems to be actively transcribed [20] , [21] . In none of these cases is there any evidence that the coding regions represent pseudogenes, and there is similarly no indication that these regions contain any transposable elements that have been completely eradicated from both genomes. For the three chromosome ends known from E. cuniculi , the corresponding E. intestinalis chromosome is missing between 11 and 16 kbp of DNA and between 9 and 11 genes ( Fig. 3 ). Moreover, in both cases in which the chromosome end is known in E. intestinalis but not in E. cuniculi , the latter can still be concluded to extend an additional 7 and 11 kbp, corresponding to five and nine genes, respectively ( Fig. 3 ). This trend seems to extend across the entire genome: in all 22 chromosome ends, E. intestinalis is truncated relative to E. cuniculi for a total of 224 kbp, corresponding to 174 genes. Interestingly, the majority of these missing genes are not recognizable homologues of any known sequence in any other organism, except E. cuniculi ( Fig. 2 ). Of these genes, 13 correspond to genes with homologues in other organisms, whereas 88 correspond to members of the DUF1609, DUF2463 or DUF1686 families, and 73 are hypothetical ORFs ( Supplementary Data 2 ). Because our assembly is gap free but 108 kbp smaller than the estimated genome size, the remaining 708 kbp difference with the genome of E. cuniculi must be due to sequences at the ends of E. cuniculi chromosomes that are absent from E. intestinalis . 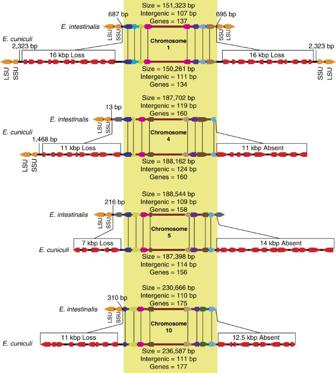Figure 3: Chromosome ends reduction inE. intestinalis. Structural comparisons between chromosomes 1, 4, 5 and 10 ofE. intestinalisandE. cuniculi. Genes and their transcriptional direction are represented by rectangular arrows. The rDNA operon linked to chromosome ends is shown in orange. Genes that are absent from theE. intestinalisassembly are shown in red, whereas genes present inE. intestinalisbut absent fromE. cuniculiare grey. The chromosome 'cores' (shaded in a yellow box) contain long blocks of absolute colinearity between the two genomes: only the first and last four orthologues in these 'cores' are shown (as coloured boxes with directional arrows) for convenience. The total size of each 'core' is indicated for both species, along with the average length of its intergenic regions and the number of genes (including tRNAs and 5S rDNAs). SSU, small subunit ribosomal RNA gene; LSU, large subunit ribosomal RNA gene. Figure 3: Chromosome ends reduction in E. intestinalis . Structural comparisons between chromosomes 1, 4, 5 and 10 of E. intestinalis and E. cuniculi . Genes and their transcriptional direction are represented by rectangular arrows. The rDNA operon linked to chromosome ends is shown in orange. Genes that are absent from the E. intestinalis assembly are shown in red, whereas genes present in E. intestinalis but absent from E. cuniculi are grey. The chromosome 'cores' (shaded in a yellow box) contain long blocks of absolute colinearity between the two genomes: only the first and last four orthologues in these 'cores' are shown (as coloured boxes with directional arrows) for convenience. The total size of each 'core' is indicated for both species, along with the average length of its intergenic regions and the number of genes (including tRNAs and 5S rDNAs). SSU, small subunit ribosomal RNA gene; LSU, large subunit ribosomal RNA gene. Full size image Conservation of non-coding sequences in Encephalitozoon spp. The significant imbalance between reduction at the chromosome ends and 'cores' suggests that the two regions are evolving under entirely different constraints. In particular, it suggests that the gene content and density of the chromosome 'cores' of both genomes have reached a certain limit. Deleterious effects of further reduction in gene content are relatively easy to imagine, as widespread gene loss presumably affects biochemical and cellular functions in an already unprecedentedly reduced proteome. The reason why the gene density has remained virtually unchanged is potentially related to the necessity of all remaining sequences to control expression. We examined this possibility by comparing sequence conservation across both genomes. Microsporidian genes are notorious for evolving very rapidly, but it is still surprising to find that the genes themselves displayed a much higher level of sequence divergence at synonymous sites than did the flanking intergenic spaces and introns ( Fig. 4 , Supplementary Table S2 and Supplementary Data 3 ). Importantly, there is no absolute correlation between the length of an intergenic space and its level of sequence conservation and, indeed, some of the longer regions are more conserved that the shortest ones (for example, the longest intergenic space in Fig. 4 ). 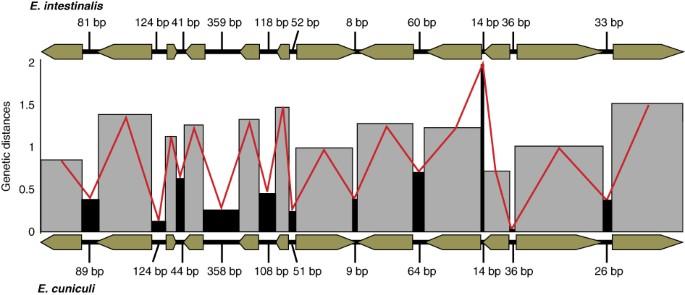Figure 4: Conservation of non-coding regions inEncephalitozoon. Schematic representation to scale of 12 orthologous genes (Ecu01_1080 to Ecu01_1170) and their intergenic spaces located on chromosome 1 ofE. intestinalis(top) andE. cuniculi(bottom). Genes and orientations are represented by rectangular olive green arrows; intergenic regions are shown in black. The scale (left) represents the genetic distance between intergenic spaces and genes (number of substitutions per synonymous site for genes, or in total for intergenic regions). Grey rectangles represent the genetic distance between genes, whereas black rectangles represent the genetic distance between intergenic regions, the progression of which is tracked by the red line. With a single exception (the 14 bp intergenic region), the intergenic spaces are always more highly conserved than the genes they surround. Figure 4: Conservation of non-coding regions in Encephalitozoon . Schematic representation to scale of 12 orthologous genes (Ecu01_1080 to Ecu01_1170) and their intergenic spaces located on chromosome 1 of E. intestinalis (top) and E. cuniculi (bottom). Genes and orientations are represented by rectangular olive green arrows; intergenic regions are shown in black. The scale (left) represents the genetic distance between intergenic spaces and genes (number of substitutions per synonymous site for genes, or in total for intergenic regions). Grey rectangles represent the genetic distance between genes, whereas black rectangles represent the genetic distance between intergenic regions, the progression of which is tracked by the red line. With a single exception (the 14 bp intergenic region), the intergenic spaces are always more highly conserved than the genes they surround. Full size image Although the E. cuniculi genome is among the smallest and most compact nuclear genomes known, the E. intestinalis genome is, at a still smaller 20%, at the known limit. By comparing the two, we can now determine which characteristics of a genome can be pushed to further extremes in these organisms, and which cannot. Although the majority of the size difference is due to gene loss, the protein-coding capacity of the two genomes is very similar because most of the genes that are absent in E. intestinalis are duplicates of genes that were retained, or unidentified ORFs. Indeed, the suite of unique genes in E. intestinalis is not only almost identical to that of E. cuniculi [3] but also scarcely different from any other known microsporidian [3] , [13] , [16] , [17] , [18] , [19] . The gene densities of E. intestinalis and E. cuniculi are also essentially the same, and the unusually high degree of conservation of intergenic sequences suggests that both genomes have also already been stripped down to a functional minimum, probably representing key regulatory elements located close to protein-coding genes in other organisms [22] , [23] . Overall, intergenic spaces and coding DNA seem to have followed similar evolutionary trajectories in maintaining what is essential for their function and getting rid of everything that is not. The contrast between these similarities and the chromosome ends is stark, but is in line with previous findings based on pulsed field gel electrophoresis and other methodologies [20] , [24] , [25] . First, genes encoded near the ends of chromosomes are known to be evolving under different pressures than are other genes [26] , [27] , and in Encephalitozoon , this is reflected by an even more elevated amino-acid sequence divergence compared with any other region of the genome. Second, these regions are known to be highly plastic in Encephalitozoon species, and characterized by frequent gene losses and gains, even between strains of one species [24] . This massive difference in coding in the subtelomeric regions does, however, raise a number of interesting questions. It is noteworthy that we do not know whether E. cuniculi or E. intestinalis better represents their common ancestral condition: it is possible that a massive expansion has taken place at the ends of E. cuniculi chromosomes or that a reduction has taken place in the E. intestinalis lineage. In either cases, the high dispensability and rapid evolution of the hypothetical genes and gene families located in those regions raise the possibility that some of these genes in extant genomes may not be functionally significant. Although there is no direct evidence that any of these genes are non-functional (and many are known to be expressed [20] ), it is possible that some of them either represent pseudogenes in the process of eroding or even spurious ORFs in the case of hypothetical ORFs. For the genes that do encode functional proteins, if the clustering of dispensable genes at chromosome ends is favoured because of the unusual conditions faced by the genes encoded there, then, paradoxically, the outright loss of these regions as in E. intestinalis would expose what were formerly 'core' genes to those conditions. Moreover, if these genes are expendable, why are they retained or even expanded in the otherwise severely compacted and reduced genome of E. cuniculi ? It is also possible or even likely that our sampling of subtelomeric region may represent only a subset of the length diversity of these highly evolving genomic regions, as the genomic template used in this study comes from a pool of over 500 million spores. We should not rule out the possibility that no single sequence adequately represents any one chromosome end of a given species because of extensive subtelomere length variation within natural populations. The identification of additional subtelomeric regions in other, intermediate-sized Encephalitozoon species and between strains of each species will provide interesting insights into the presence of potential variation at these unusually evolving genomic regions, and also a miniature view of how different pressures shape different regions of nuclear genomes in general. Cultivation and collection of E. intestinalis material Spores from E. intestinalis (ATCC 50506; originally isolated from human alveolar lavage) were grown in the rabbit kidney fibroblast cell line, RK 13 (ATCC CCL-37), with RPMI 1640 supplemented with 5% fetal bovine serum, 2 mM L -glutamine and antibiotics (100 U penicillin per ml, 100 μg streptomycin per ml). T75 flasks were incubated at 37 °C with 5% CO 2 , and culture medium was replaced two or three times per week. Supernatants containing spores were stored at 4 °C until extraction of DNA. To enrich spores from host cell debris, the collected culture supernatants were subjected to sequential washes at 400 g each with distilled H 2 O, TBS-Tween 20 (0.3%) and Tris buffered saline (TBS). The final pellet was then resuspended in TBS and mixed with an equal volume of 100% Percoll, followed by centrifugation at 400 g for 45 min at 4 °C. Host cell debris in the top 75% volume of Percoll was removed. The lower 25% volume of Percoll and the pellet were then transferred to a new tube, resuspended in TBS and washed several times. Owing to continued adherence of host cell (that is, rabbit) nucleic acid onto the spores, an additional series of washes were performed with TBS-SDS (0.1%), followed by three washes with TBS. DNA extraction procedure Genomic DNA was extracted from approximately 500 million spores. Spores were pelleted by centrifugation, resuspended in 300 μl of lysis solution (EPICENTRE Biotechnologies) containing Proteinase K and mixed thoroughly using a vortex. Glass beads (200 μl, 150–212 μm in diameter) were added to the sample, which was immediately incubated at 65 °C for 15 min and bead-beaten at 2,500 r.p.m. for 30 s every 5 min. The sample was then cooled to 37 °C and incubated for 30 min at the same temperature on addition of 2 μl of 5 μg μl −1 RNase A. After treatment with RNAse, the sample was placed on ice for 5 min, 150 μl of MPC Protein Precipitation Reagent (EPICENTRE Biotechnologies) was added and the solution was vortexed vigorously for 10 s. Protein debris was pelleted at 4 °C for 10 min at a speed of ≥10,000 g and the supernatant was transferred to a clean microcentrifuge tube. DNA was then precipitated using isopropanol, rinsed twice using 70% ethanol and the DNA was finally suspended in TE buffer. Genome sequencing and de novo assembly For deep sequencing, a genomic shotgun library was prepared from less than 200 ng of genomic DNA. We used Fasteris-modified bar-coded adapters to permit multiplexing, in this case using an ACTGT bar code at the beginning of the forward and reverse reads. Fragments with inserts of approximately 320–340 bp were selected, and an aliquot of the library was cloned into a TOPO plasmid and seven clones were sequenced by Sanger to confirm for insert sizes and that the constructs were derived from Encephalitozoon . The library was then subjected to deep sequencing using half a channel of the Illumina GAIIx instrument and 31 bp paired-end reads (with an average insert of 337 bp), resulting in 428,131,080 bp of unique DNA sequence. Reads were assembled using Velvet [29] with a hash value of 19, resulting in 137 scaffolds with an average size of 16,181 bp and an average coverage of 40×. Genome completion and annotation and analysis PCR using nested primers, cloning and Sanger sequencing were used in combination with Consed [29] to validate the breaks within the scaffolds and to link scaffold together into 11 continuous sequences homologous to the 11 chromosomes of E. cuniculi . Subtelomeric regions were obtained using nested PCR and Sanger sequencing, with forward primers designed on large subunit ribosomal RNA of E. intestinalis in combination with primers designed on the first and last identifiable genes from the 'core' of each chromosome. We define the chromosomal 'cores' heuristically as the genomic sequence located between the first and last recognizable E. intestinalis gene that has a clearly recognizable orthologue in E. cuniculi . Other chromosomal locations are referred to as 'subtelomeric' regions. Annotation was manually performed using Artemis [30] in combination with BLAST procedures [31] against the genome of E. cuniculi and the 'non-redundant' repository at NCBI. Transfer RNAs were detected using tRNAscan-SE [32] and spliceosomal introns were manually detected. Pairwise genetic distances between orthologous intergenic sequences of E. intestinalis and E. cuniculi were calculated using the maximum likelihood methodology implemented in MEGA4. [33] Pairwise genetic distances between fourfold degenerate (neutral) sites of orthologous genes were calculated using the Kumar method. [33] Sequences of the 11 individual E. intestinalis chromosomes are available from GenBank under accession numbers CP001942 , CP001943 , CP001944 , CP001945 , CP001946 , CP001947 , CP001948 , CP001949 , CP001950 , CP001951 and CP001952 . How to cite this article: Corradi, N. et al . The complete sequence of the smallest known nuclear genome from the microsporidian Encephalitozoon intestinalis . Nat. Commun. 1:77 doi: 10.1038/ncomms1082 (2010).